Bio-responsive polymer hydrogels homeostatically regulate blood coagulation Bio-responsive polymer architectures can empower medical therapies by engaging molecular feedback-response mechanisms resembling the homeostatic adaptation of living tissues to varying environmental constraints. Here we show that a blood coagulation-responsive hydrogel system can deliver heparin in amounts triggered by the environmental levels of thrombin, the key enzyme of the coagulation cascade, which—in turn—becomes inactivated due to released heparin. The bio-responsive hydrogel quantitatively quenches blood coagulation over several hours in the presence of pro-coagulant stimuli and during repeated incubation with fresh, non-anticoagulated blood. These features enable the introduced material to provide sustainable, autoregulated anticoagulation, addressing a key challenge of many medical therapies. Beyond that, the explored concept may facilitate the development of materials that allow the effective and controlled application of drugs and biomolecules. Implementing biomolecular recognition in synthetic materials has enabled a wealth of applications with examples ranging from engineered extracellular matrices over targeted drug delivery to highly selective molecular sensors. However, almost all of the related systems are limited by the fact that bioactivity is pre-defined or uni-directionally adjusted by simple adaptation schemes—based on, for example, changes in pH, temperature or enzymatic activity [1] , [2] , [3] , [4] , [5] , [6] , [7] , [8] , [9] —which are often highly useful, for example in site-targeted drug delivery [10] but cannot afford feedback regulation. In contrast, living organisms employ an arsenal of robust molecular mechanisms that maintain homeostasis and enable precisely adjusted functionality under varying environmental settings. Examples comprise processes constituting tissue development and repair, immune response and blood coagulation. As many of the involved homeostatic effector-inhibitor pairs have now been thoroughly analysed (for example, the regulation of the blood glucose level by insulin and glucagon, or the control over immune response and autoimmunity by regulatory T cells, and several others), recapitulating bi-directionally coupled molecular ‘if-then-functions’ in engineered materials and systems holds great promise for tailoring medical interventions to match spatiotemporally varying needs. However, only few feedback-controlled bio-responsive delivery systems have been developed so far, with insulin release materials responding to the blood glucose concentration being the most prominent group [11] , [12] , [13] . Offering unprecedented options for adjusting the release profile, the regulation loop in this system is rather complex and requires the response of the living organism as a whole [14] . Going clearly beyond those earlier reports, we suggest here a direct feedback loop system with immediate effect of the response (heparin release) to the trigger (thrombin level). The approach is based on well-known molecular components, addressing a prevalent problem associated with the application of many current medical devices and therapies: the undesired activation of blood coagulation. Blood coagulation is a cascade process resulting in clot formation preventing blood loss and enabling the repair of damaged blood vessels. This protective mechanism can, however, backfire with potentially fatal consequences when triggered inopportunely such as the formation of thromboses or emboli in response to applying medical devices like the cardiopulmonary bypass [15] , [16] , [17] , [18] , [19] . The mucopolysaccharide heparin is routinely administered clinically to counteract coagulation activation [20] , [21] . Thrombin, the key enzyme of the coagulation cascade, binds heparin when activated. The natural thrombin inhibitor, antithrombin, also has a heparin-binding site recognizing a pentasaccharide sequence on heparin to which it binds immobile. Thrombin has no such sequence specificity and can slide along the heparin chain where it associates with antithrombin to form a covalent enzyme inhibitor complex that subsequently dissociates from heparin [22] . As systemic use of heparin remains difficult to regulate, causing a significant risk of under- or overdosage, both associated with dangerous consequences, the immobilization of heparin to surfaces has been explored for blood contacting materials used in medical devices [18] , [23] , [24] with end-grafted heparin layers currently being clinically favored and routinely applied [18] , [19] . Despite the resulting benefits, the protective effect of heparin-containing coatings is obviously limited due to the invariant, rather low amounts of anticoagulant and restrictions of its accessibility. Therefore, the controlled release of anticoagulant agents such as heparin receives growing interest [23] , [25] . Conventional release concepts are, however, inappropriate as the released quantities have to match the actual levels of coagulation activation permanently, which can rapidly and drastically change due to amplification effects. Consequently, the only current option is overdosage of anticoagulant as the lesser evil. This challenge provides an ideal model system to address using an engineered feedback-controlled delivery system. To this end, we present a modular hydrogel consisting of heparin and multi-armed poly(ethylene glycol) (starPEG) covalently linked by peptide units that contain the sequence (D)Phe-Pip-Arg-Ser, which is cleaved by thrombin after arginine with high selectivity [26] . As illustrated in Fig. 1 , thrombin formation results in the cleavage of the gel and in the release of heparin. Together with the subsequent complexation of heparin-bound thrombin and antithrombin, this creates a control loop system, where the response, that is, release of heparin, downregulates the trigger, the activated coagulation cascade. Thus, the newly developed bio-responsive polymer hydrogels can turn enemy into friend; making thrombin, the key factor of the coagulation, a switch that sensitively regulates anticoagulation. The introduced material is demonstrated to suppress human whole-blood coagulation for several hours even in presence of a pro-coagulant surface. A blood resupply experiment shows the durability of the bio-responsive characteristics of the hydrogels and confirms their advantage over non-responsive heparinized reference materials. 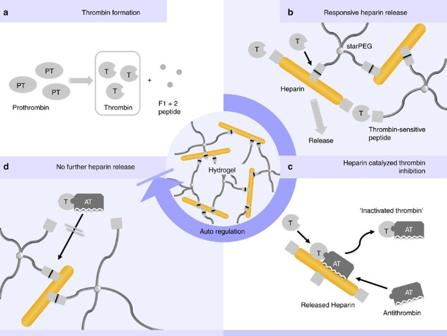Figure 1: Autoregulation of heparin release from thrombin-sensitive starPEG-heparin hydrogels. (a) Thrombin generation from prothrombin, as caused by various different activation schemes associated with the exposure of blood to foreign materials, carries the risk of subsequent thrombus formation. (b) As a selective protease, thrombin cleaves the peptide NH2-Gly-Gly-(D)Phe-Pip-Arg-Ser-Trp-Gly-Cys-Gly-CONH2of the linker unit in the biohybrid starPEG-heparin materials between arginine and serine. Through this, heparin becomes released with kinetics that depend on the degree of crosslinking. (c) Released heparin catalyses the complexation of thrombin with its plasma-based inhibitor, antithrombin, resulting in the inactivation of thrombin. (d) Removal of thrombin from the system according to (c) terminates gel degradation and further heparin release. Figure 1: Autoregulation of heparin release from thrombin-sensitive starPEG-heparin hydrogels. ( a ) Thrombin generation from prothrombin, as caused by various different activation schemes associated with the exposure of blood to foreign materials, carries the risk of subsequent thrombus formation. ( b ) As a selective protease, thrombin cleaves the peptide NH 2 -Gly-Gly-(D)Phe-Pip-Arg-Ser-Trp-Gly-Cys-Gly-CONH 2 of the linker unit in the biohybrid starPEG-heparin materials between arginine and serine. Through this, heparin becomes released with kinetics that depend on the degree of crosslinking. ( c ) Released heparin catalyses the complexation of thrombin with its plasma-based inhibitor, antithrombin, resulting in the inactivation of thrombin. ( d ) Removal of thrombin from the system according to ( c ) terminates gel degradation and further heparin release. Full size image Preparation of thrombin-responsive hydrogels The gels were prepared by conversion of activated carboxylic acid groups of heparin with the N-termini of thrombin-responsive NH 2 -Gly-Gly-(D)Phe-Pip-Arg-Ser-Trp-Gly-Cys-Gly-CONH 2 peptides that were conjugated before to maleimide terminated starPEG molecules through the cystein moiety. Non-responsive reference materials were either obtained by direct conjugation of the N-terminated starPEG to the activated carboxylic groups of heparin or by applying a scrambled sequence of the thrombin-responsive peptide where the P2 amino acid Pip and the P1’ amino acid Ser were exchanged. Structural considerations of the binding pocket of thrombin and physiological thrombin substrates suggest that this sequence warrants stability against cleavage by this particular protease [27] . As heparin has multiple carboxylic acid moieties the degree of crosslinking (CL) of the gel networks can be adjusted by varying the ratio of the reactive building blocks. Hydrogels similarly made of heparin and starPEG were previously shown to allow for an independent modulation of network structure (that is, elasticity, meshsize and hydration) and heparin concentration [28] , [29] . Thus, the accessibility for soluble proteins can be varied for sets of these gels with invariant heparin content. To verify the thrombin-responsive degradation, gels with different CL degree (low, medium and high CL degree, see Supplementary Fig. S1 ) were exposed to thrombin solutions and the heparin release was quantified ( Fig. 2a ). All gels were found to release heparin as a function of the thrombin concentration, and the degradation rates were decreased in the higher crosslinked gels. Heparin release rates were observed to be linear without any initial burst release nor lag phase, ensuring a precisely adjusted and immediate anticoagulant response of the hydrogel to elevated environmental thrombin levels. The release covered very well previously estimated rates of 2.4 μg cm −2 h −1 required for an anticoagulant microenvironment [25] . The heparin release from the hydrogels linked through scrambled peptides was only about 4% of the thrombin-responsive hydrogel, indicating resistance to cleavage by thrombin. The scrambled-peptide reference hydrogels also showed substantially reduced heparin release when exposed to whole blood, which contains a number of non-specific proteases ( Fig. 2b ). 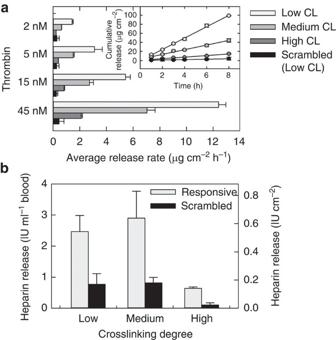Figure 2: Heparin release rate from thrombin-responsive starPEG-heparin hydrogels. (a) Hydrogels containing the thrombin-cleavable crosslinker NH2-Gly-Gly-(D)Phe-Pip-Arg-Ser-Trp-Gly-Cys-Gly-CONH2.with low, medium and high degrees of CL or the scrambled sequence NH2-Gly-Gly-(D)Phe-Ser-Arg-Pip-Trp-Gly-Cys-Gly-CONH2with low degree of CL (characterized by storage moduli of 3, 8, and 16 kPa, respectively, seeSupplementary Fig. S1) were prepared to contain 1% Alexa 488 conjugated heparin. The gels were incubated with 170 μl cm−2Tris-BSA-buffer solution of varied thrombin concentration. At various points of time, the released heparin concentration in the supernatant was determined by fluorescence measurement. The heparin release is linear with time (inset) and shows a clear correlation with both the degree of CL of the gels and the thrombin concentration of the solution. (mean±s.d.,n=3) (b) The sets of hydrogels crosslinked with the responsive or scrambled peptide sequence at the different degrees of CL were incubated with 1 U ml−1heparinized whole blood for 3 h. After the incubation, the heparin concentration was determined in a FXa-based activity assay and corrected for the baseline anticoagulation. The heparin release from gels containing the scrambled-peptide sequence was reduced to 10–30% of the release from gels containing thrombin-cleavable peptide linkers. (mean±s.d.,n=6). Figure 2: Heparin release rate from thrombin-responsive starPEG-heparin hydrogels. ( a ) Hydrogels containing the thrombin-cleavable crosslinker NH 2 -Gly-Gly-(D)Phe-Pip-Arg-Ser-Trp-Gly-Cys-Gly-CONH 2 .with low, medium and high degrees of CL or the scrambled sequence NH 2 -Gly-Gly-(D)Phe-Ser-Arg-Pip-Trp-Gly-Cys-Gly-CONH 2 with low degree of CL (characterized by storage moduli of 3, 8, and 16 kPa, respectively, see Supplementary Fig. S1 ) were prepared to contain 1% Alexa 488 conjugated heparin. The gels were incubated with 170 μl cm −2 Tris-BSA-buffer solution of varied thrombin concentration. At various points of time, the released heparin concentration in the supernatant was determined by fluorescence measurement. The heparin release is linear with time (inset) and shows a clear correlation with both the degree of CL of the gels and the thrombin concentration of the solution. (mean±s.d., n =3) ( b ) The sets of hydrogels crosslinked with the responsive or scrambled peptide sequence at the different degrees of CL were incubated with 1 U ml −1 heparinized whole blood for 3 h. After the incubation, the heparin concentration was determined in a FXa-based activity assay and corrected for the baseline anticoagulation. The heparin release from gels containing the scrambled-peptide sequence was reduced to 10–30% of the release from gels containing thrombin-cleavable peptide linkers. (mean±s.d., n =6). Full size image Hydrogel performance in whole-blood incubation Next, the thrombin-responsive hydrogels—and a corresponding set of non-responsive gels for comparison—were exposed for 3 h to freshly drawn human whole blood in well-defined incubation assays [30] . The heparin released into plasma from the degraded gels is shown in Fig. 3a (anti FXa units, related to the blood volume and to the gel surface); there was no release from the non-responsive gels. In line with the heparin release data obtained upon incubation in the thrombin solutions ( Fig. 2 ), the release rate depended on the CL degree of the gel. Thrombin formation was determined via the F1+2 peptide, which is cleaved off prothrombin during activation. Heparin released from the thrombin-responsive gels resulted in an additional anticoagulant effect when compared with the corresponding non-responsive starPEG-heparin gels ( Fig. 3b ). The anticoagulant effect clearly correlated with the amounts of heparin released and the related degree of gel CL. As thrombin is a main activator of blood platelets, platelet activation was true to the levels of thrombin formation ( Fig. 3c ). Neither the non-responsive nor the thrombin-responsive gels caused critical levels of inflammatory response as measured by the complement system (for details see Supplementary Fig. S2 ). 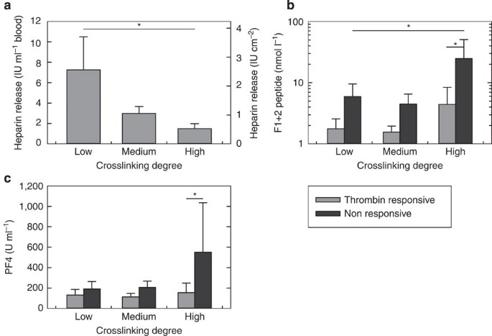Figure 3: Whole-blood incubation with thrombin-responsive and non-responsive gels. Gels with low, medium and high degrees of CL (storage moduli of 3, 8 and 16 kPa respectively, seeSupplementary Fig. S1) on glass supports were incubated with freshly drawn human whole blood at a ratio of 2 ml blood per 6.3 cm2gel surface area for 3 h. (a) Heparin release during the incubation. The heparin release from the gels with thrombin-cleavable sequence correlated strongly with the degree of CL. These released heparin concentrations reach pharmacologically relevant levels. All heparin release was through enzymatic degradation of the peptide crosslinker, as no heparin was released from the gels without that linker. (b) F1+2 peptide and (c) platelet factor 4 release were determined in plasma by ELISA and reflect plasmatic coagulation activation and platelet activation, respectively. The elevated plasmatic heparin concentrations produced by the cleavable gels enhanced their thromboresistant properties, seen as decreased thrombin formation (F1+2 peptide) and platelet response. (mean±s.d.,n=6 in all panels; asterisks indicateP<0.05 in analysis of variance (ANOVA) with Student–Newman–Keulspost-hocanalysis). Figure 3: Whole-blood incubation with thrombin-responsive and non-responsive gels. Gels with low, medium and high degrees of CL (storage moduli of 3, 8 and 16 kPa respectively, see Supplementary Fig. S1 ) on glass supports were incubated with freshly drawn human whole blood at a ratio of 2 ml blood per 6.3 cm 2 gel surface area for 3 h. ( a ) Heparin release during the incubation. The heparin release from the gels with thrombin-cleavable sequence correlated strongly with the degree of CL. These released heparin concentrations reach pharmacologically relevant levels. All heparin release was through enzymatic degradation of the peptide crosslinker, as no heparin was released from the gels without that linker. ( b ) F1+2 peptide and ( c ) platelet factor 4 release were determined in plasma by ELISA and reflect plasmatic coagulation activation and platelet activation, respectively. The elevated plasmatic heparin concentrations produced by the cleavable gels enhanced their thromboresistant properties, seen as decreased thrombin formation (F1+2 peptide) and platelet response. (mean±s.d., n =6 in all panels; asterisks indicate P <0.05 in analysis of variance (ANOVA) with Student–Newman–Keuls post-hoc analysis). Full size image Response of hydrogels to challenging conditions The coagulation activation levels of thrombin-responsive versus non-responsive gels reported in Fig. 3 clearly show the impact of released heparin as it is dependent on the thrombin levels and CL of the gels, proving the additional protective effect resulting from the incorporation of thrombin-cleavable peptide units. As expected, coagulation activation with the heparin-containing gel materials as the only foreign surface remained rather low in general, evoking the question of the capability of the cleavable gels to passivate additional activation events remote from the gel. To assess this, whole blood was simultaneously exposed to two different surfaces on either side of the incubation chambers: a thrombin-responsive (or a reference with the non-responsive scrambled sequence) gel layer and a second surface with known activation effect on the blood coagulation. The latter surface consisted of binary self-assembled monolayers of carboxylic acid- and methyl terminated alkane thiols on gold, which produce activation levels dependent on the content of terminating carboxylic acid groups [24] . For all investigated systems, coagulation activation was more effectively prevented in co-incubation with the thrombin-responsive gels than with the non-responsive reference containing a scrambled-peptide sequence. This effect was most prominent in the presence of a highly pro-coagulant 85%-COOH surface ( P <0.01, analysis of variance with Student–Newman–Keuls post-hoc analysis) ( Fig. 4 ), confirming the expectation that the feedback-controlled materials can quench coagulation activation occurring remote of the hydrogel-coated surfaces. 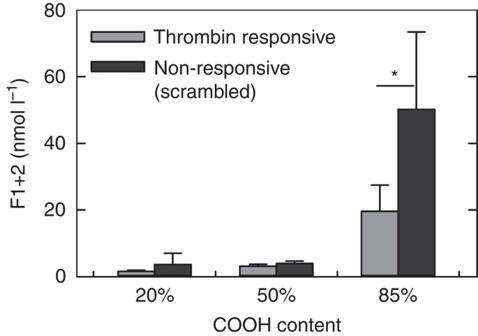Figure 4: Anticoagulant capacity of starPEG-heparin gels in presence of a second surface with graded coagulation activation potential. Whole blood was co-incubated for 3 h with thrombin-responsive or non-responsive gels containing the scrambled-peptide sequence (low degree of CL, 3 kPa) and a set of binary self-assembled monolayers of carboxylic acid- and methyl-terminated alkane thiols. (The composition of the self-assembled monolayers was varied to modulate the activation level according to (24)). Both the non-responsive and the thrombin-responsive gels compensated the coagulation activation by weakly and intermediately activating surfaces. However, in presence of a highly pro-coagulant self-assembled monolayer, thrombin-responsive gels were capable of maintaining a low coagulation level, whereas elevated coagulation activation and blood clot formation occurred with the non-cleavable reference gel under otherwise similar conditions (P<0.01, ANOVA with Student–Newman–Keulspost-hocanalysis). (mean±s.d.,n=6). Figure 4: Anticoagulant capacity of starPEG-heparin gels in presence of a second surface with graded coagulation activation potential. Whole blood was co-incubated for 3 h with thrombin-responsive or non-responsive gels containing the scrambled-peptide sequence (low degree of CL, 3 kPa) and a set of binary self-assembled monolayers of carboxylic acid- and methyl-terminated alkane thiols. (The composition of the self-assembled monolayers was varied to modulate the activation level according to (24)). Both the non-responsive and the thrombin-responsive gels compensated the coagulation activation by weakly and intermediately activating surfaces. However, in presence of a highly pro-coagulant self-assembled monolayer, thrombin-responsive gels were capable of maintaining a low coagulation level, whereas elevated coagulation activation and blood clot formation occurred with the non-cleavable reference gel under otherwise similar conditions ( P <0.01, ANOVA with Student–Newman–Keuls post-hoc analysis). (mean±s.d., n =6). Full size image Encouraged by these findings we furthermore exposed the gel materials and clinically applied vascular grafts made of expanded poly(tetrafluoroethylene), with or without endpoint-attached heparin coatings, to freshly drawn whole blood without any soluble anticoagulant added. In the presence of thrombin-responsive hydrogels, blood was protected from clotting over the whole investigated time period of 1 h, whereas blood in contact with the non-responsive gels or the clinically applied materials completely coagulated under these conditions ( Fig. 5 ). Accordingly, prothrombin F1+2 fragment concentration drastically differed in between the responsive and non-responsive materials. After 1 h of incubation with blood, we replaced the blood and exposed the surfaces for another hour to fresh blood under the same conditions to test the possible exhaustion of the thromboresistant effect of the compared samples. Referring to the comprehensive studies by K.G. Mann et al . [31] , [32] , [33] , the implemented ‘resupply experiment’ is considered to realistically simulate the conditions of blood flow: In the second incubation cycle, fresh blood containing the full set of non-activated coagulation factors is exposed to hydrogel surfaces which retain adsorbed, activated clotting factors from the previous incubation cycle. Upon the second exposure, blood in contact with the thrombin-responsive hydrogels again remained liquid, whereas blood on all the other surfaces coagulated. This observation was underpinned by the measured F1+2 fragment formation ( Fig. 5 ), showing similarly high values for all non-responsive surfaces and significantly lower levels for the thrombin-responsive hydrogels. 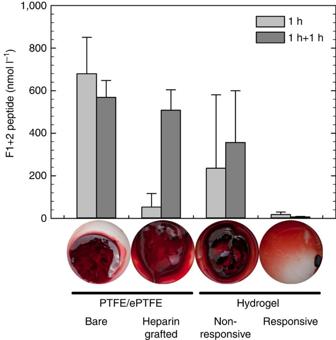Figure 5: Whole-blood incubation with blood exchange. Clinically applied polytetrafluoroethylene (vascular graft) materials with and without endpoint-immobilized heparin, non-responsive and thrombin-responsive starPEG-heparin materials were incubated with whole blood. After 1 h, the blood volume was replaced against fresh blood and the samples were incubated once again for 1 h. No anticoagulant was added to the blood. Concentrations of the prothrombin F1+2 fragment after the incubation periods indicate that only thrombin-responsive gels effectively suppress the thrombin generation loop (P<0.05 versus all controls by ANOVA with Student–Newman–Keulspost-hocanalysis). Upon the second incubation with fresh blood, applied to probe for the possible exhaustion of the coatings, the anticoagulant effect of the responsive gel was fully maintained (P<0.05 versus all controls by ANOVA with Student–Newman–Keulspost-hocanalysis), whereas the endpoint-attached heparin surface lost activity. (Bars present mean±s.d.,n=9) Bottom: The blood remained liquid with the thrombin-responsive gels (right) during an incubation period of 3 h. In contrast, a solid blood clot was formed on the non-responsive gels, the end-grafted heparin coating and the bare polytetrafluoroethylene surface over the same time period. Figure 5: Whole-blood incubation with blood exchange. Clinically applied polytetrafluoroethylene (vascular graft) materials with and without endpoint-immobilized heparin, non-responsive and thrombin-responsive starPEG-heparin materials were incubated with whole blood. After 1 h, the blood volume was replaced against fresh blood and the samples were incubated once again for 1 h. No anticoagulant was added to the blood. Concentrations of the prothrombin F1+2 fragment after the incubation periods indicate that only thrombin-responsive gels effectively suppress the thrombin generation loop ( P <0.05 versus all controls by ANOVA with Student–Newman–Keuls post-hoc analysis). Upon the second incubation with fresh blood, applied to probe for the possible exhaustion of the coatings, the anticoagulant effect of the responsive gel was fully maintained ( P <0.05 versus all controls by ANOVA with Student–Newman–Keuls post-hoc analysis), whereas the endpoint-attached heparin surface lost activity. (Bars present mean±s.d., n =9) Bottom: The blood remained liquid with the thrombin-responsive gels (right) during an incubation period of 3 h. In contrast, a solid blood clot was formed on the non-responsive gels, the end-grafted heparin coating and the bare polytetrafluoroethylene surface over the same time period. Full size image A number of recently described functional hydrogel systems utilized the responsiveness of polymers to various biomolecules. Biomimicry concepts relying on bio-adaptive polymeric components were, for example, successfully employed in the design of cell-responsive polymer matrix materials for tissue engineering, drug release systems and sensory devices [1] , [2] , [3] , [4] , [5] , [6] , [7] , [8] , [9] , [10] . However, the response of the material in these systems affects the trigger indirectly through multistep physiological interactions. The thrombin-responsive gel material introduced here conceptually goes beyond by producing a molecular signal (that is, the release of heparin) that directly modulates its biomolecular trigger (thrombin) without need for any additional effectors. This makes the approach clearly advantageous for protective coatings of blood contacting medical devices with self-adjusted, localized administration of the anticoagulant and avoiding the bleeding hazard of high-dose systemic anticoagulation. Immobilized thrombin-responsive hydrogel layers were found to be stable upon whole-blood incubation and during storage in aqueous media without any signs of fragmentation or delamination ( Supplementary Fig. S3 ). Given the adjustable volume and degree of CL of the gel coatings, protection can be maintained over periods of several days at elevated thrombin levels (assuming a constant release of 2.4 μg cm −2 h −1 (ref. 25 )) and several months at physiological baseline thrombin concentrations (1–10 nmol l −1 ) [34] . Thus, the developed material not only outperforms currently applied anticoagulant coatings over shorter time periods, but can be anticipated to offer a ‘silent’ long-term protection due to its thrombin-responsive heparin release through a self-renewing surface. The resupply experiment, avoiding a steady pool effect by replacing the blood after 1 h, provided data that suggest the explored concept to be effective under conditions of blood flow in vivo , which has to be experimentally verified in further studies. As the main components of the introduced gel materials are already medically approved and widely used, the described system is considered attractive for clinical translation. Similar bio-responsive gels with sensitivity to the more upstream coagulation factor FXa or delivery of direct—synthetic—coagulation inhibitors instead of heparin offer promising variations of the introduced design concept [35] . In conclusion, the reported system is a simple yet powerful and clinically relevant example illustrating the enormous potential of reciprocally triggered bio-responsive polymers. Exploiting this new paradigm seems particularly attractive for the auto-adjusted administration of drugs and bioactives along various therapeutic avenues. Further developments may adapt the principle of bi-directionally coupled molecular ‘if-then-functions’ in materials to aid regenerative therapies by providing morphogenic signals in dependence on the progress of tissue formation. Similarly, such feedback-controlled materials may pave the way for truly autonomous functional compartments in synthetic biology. Peptide synthesis The sequence (D)F-Pip-RS was included as a bioactive motif into the peptide NH 2 -GG-(D)F-Pip-RSWGCG-CONH 2 (FXRS), where Pip abbreviation stands for (R)-pipecolic acid and (D)F is D -phenyl alanine. The peptide was synthesized by standard Fmoc solid-phase techniques on an amide resin and its purity was confirmed by analytical high-performance liquid chromatography and electrospray ionization mass spectrometry (for details see Supplementary Methods ). Synthesis of the polyethylene glycol (PEG)-peptide (PEG-FXRS) conjugate was performed by stoichiometric reaction between the thiol group of cysteine and the terminal maleimide groups of starPEG (MW 10,000, JenKem Technology USA Inc (Allen, USA)) as previously described with a conversion rate above 90% [36] . As shown by the RGD sequence [37] example the guanidinium group of arginine does not participate in the formation of such PEG-peptide conjugates or 1-ethyl-3-(3-dimethylaminopropyl) carbodiimide/ N -hydroxysulfosuccinimide (NHS) reaction that is later utilized to form the gel network with heparin. Therefore, PEG-FXRS conjugate was expected to keep the biological activity of the apopeptide in the proposed gel material. Gel preparation Unmodified amino-terminated starPEG or the peptide functionalized starPEG (PEG-FXRS) were used for formation of non-responsive or thrombin-responsive hydrogels, respectively. Heparin (MW 14,000, Merck, Germany) activation was done using 1-ethyl-3-(3-dimethylaminopropyl) carbodiimide and sulfo-NHS (ratio 2:1) at a stoichiometric balanced concentration of sulfo-NHS to the starPEG-NH 2 -groups for 15 min on ice. Then starPEG (MW 10,000, JenKem) or the starPEG peptide conjugates (PEG-FXRS or the scrambled sequence PEG-FSRX) was added at the starPEG: heparin stoichiometry according to the gel type. Low (G′≈3 kPa), medium (G′≈8 kPa) and high (G′≈16 kPa) degrees of CL were obtained in non-cleavable and thrombin-responsive gels prepared from molar ratios of 2:1, 3:1, 6:1 and 0.75:1, 1:1, 2:1, respectively. (Differences in reactivity of the components were compensated by adjusting their molar ratios to create gels with similar storage moduli (see Supplementary Fig. S1 ) and accordingly similar CL degrees). The gel-forming components in each mixture added up to 133 mg ml −1 . The mixture was evenly spread on poly(ethylene) alt maleic anhydride co-polymer-coated glass supports [38] as 10 μl cm −2 gel solution per surface and covered with Sigmacote hydrophobized glass disks. After overnight polymerization, the cover disks were removed and the hydrogels were swollen to about 70 μm and repeatedly washed in phosphate buffered saline (PBS) for 24 h. Heparin release from degradable gels Gels were prepared where 1% of the heparin was substituted by Alexa 488 (Molecular Probes/Invitrogen, Darmstadt, Germany) conjugated heparin. Gel disks (1.55 cm 2 ) were equilibrated in Tris-BSA-buffer (100 mM NaCl, 50 mM tris(hydroxymethyl)aminomethane, 0.1% bovine serum albumin, pH 7.4) and then immersed in 200 μl thrombin at the given concentrations in Tris-BSA-buffer. The heparin concentration in the supernatant was determined by measuring the released fluorescence in a microplate reader (Tecan Genios, Tecan Ltd, Männedorf, Switzerland) and calibration with a standard curve of defined concentrations. Self-assembled monolayers of alkylthiols The process of self-assembled monolayers preparation is described in detail elsewhere [24] . Briefly, an 80 nm gold layer was evaporated on glass disks with a connecting layer of 3 nm chromium. The gold layer was immersed for 20 min in 0.2 mM alkanethiol solutions in tetrahydrofuran, composed of the desired ratios of 11-mercaptoundecanoic-acid (-COOH) and undecanethiol (-CH 3 ), rinsed with tetrahydrofuran and ethanol and dried in a stream of nitrogen. Whole-blood incubation The method has been described in detail elsewhere [30] . Briefly, freshly drawn venous blood from two AB0 compatible donors after obtaining informed consent, free from medication for the preceeding 10 days, was immediately low dose anticoagulated with 1.0 U ml −1 heparin unless otherwise stated, and pooled. The hydrogel samples and SAM surfaces on glass supports were applied as top and bottom of in house designed incubation chambers, in which 2 ml blood contact 6.3 cm 2 test surface and 4 cm 2 chamber material PTFE. Reference materials for the application-oriented two-stage blood incubation experiment were commercial vascular grafts of expanded poly(tetrafluoroethylene) with or without endpoint-attached heparin (GORE PROPATEN, Carmeda BioActive surface or GORE-TEX, respectively). The incubation was performed at 37 °C under constant revolution and avoiding air contact for 3 h. ELISA tests using commercial kits for thrombin F1+2 fragment (Dade Behring/Siemens, Marburg, Germany) and platelet factor 4 (Haemochrom, South Bend, Il) were performed after the incubation period. The heparin concentration was determined using a chromogenic factor Xa-based test kit (Chromogenix, Milano, Italy). The study has been approved by the Ethics Committee of the Sächsische Landesärztekammer, Dresden, Germany. Statistical assessment All blood incubations were performed twice with different donors and triplicate sets of samples in parallel ( n =6, 4 blood donations). Other analyses were performed at least in triplicate. Data are presented as mean and s.d.. Tests for statistical significance were performed by analysis of variance with a multiple comparisons procedure according to Student–Newman–Keuls (SigmaPlot 12.3, Systat). Differences with P <0.05 are considered statistically significant and are indicated by an asterisk in the Figures. How to cite this article: Maitz, M. F. et al . Bio-responsive polymer hydrogels homeostatically regulate blood coagulation. Nat. Commun. 4:2168 doi: 10.1038/ncomms3168 (2013).